Unidirectional suppression of hydrogen oxidation on oxidized platinum clusters Solar-driven water splitting to produce hydrogen may be an ideal solution for global energy and environment issues. Among the various photocatalytic systems, platinum has been widely used to co-catalyse the reduction of protons in water for hydrogen evolution. However, the undesirable hydrogen oxidation reaction can also be readily catalysed by metallic platinum, which limits the solar energy conversion efficiency in artificial photosynthesis. Here we report that the unidirectional suppression of hydrogen oxidation in photocatalytic water splitting can be fulfilled by controlling the valence state of platinum; this platinum-based cocatalyst in a higher oxidation state can act as an efficient hydrogen evolution site while suppressing the undesirable hydrogen back-oxidation. The findings in this work may pave the way for developing other high-efficientcy platinum-based catalysts for photocatalysis, photoelectrochemistry, fuel cells and water–gas shift reactions. Photocatalytic water splitting is a process for potentially green and renewable hydrogen generation [1] , [2] , [3] , [4] . Over the past decades, many revolutionary photocatalysts have been developed, and most of them require cocatalysts to act as active sites for H 2 evolution at their surface [5] , [6] , [7] , [8] , [9] . To date, various noble metals and semiconductors have been used to cocatalyze water decomposition into hydrogen and oxygen [10] , and in particular, metallic platinum nanoparticles (m-Pt NPs) have been widely employed as the cocatalyst with various light-harvesting semiconductors for the hydrogen evolution reaction (HER) [11] . In a photocatalytic system modified with m-Pt NPs cocatalyst, the photoexcited electrons in semiconductors can rapidly transfer to the m-Pt NPs cocatalysts through the metal–semiconductor interface (Schottky layer), and reduce protons (H + ) in an aqueous reaction medium to form H 2 (ref. 12 ). Unfortunately, hydrogen back-oxidation is also catalysed by metallic Pt cocatalysts because of their robust adsorption property and its low activation energy [13] . This is a classical reaction applied in the proton exchange membrane fuel cell that can convert chemical energy directly into electrical energy [14] . This undesirable back-reaction drastically limits the solar energy conversion efficiency of fuel-reforming catalysts, and it is an open challenge to specifically suppress the undesirable hydrogen oxidation reaction (HOR) while preserving an efficient hydrogen evolution rate in artificial photosynthesis systems [15] , [16] . Here we find that Pt in a higher oxidation state (that is, PtO) demonstrates remarkable HOR suppression ability, while its hydrogen evolution capacity is still comparable to that of the benchmark of conventional metallic Pt cocatalyst through comprehensive experimental and theoretical analysis (see Fig. 1 for schematic mechanism). This work confirms the role of PtO cocatalyst in governing the preferred direction of H 2 reactions, and the finding may pave the way for developing other high-efficientcy catalysts for water splitting, water–gas shift reactions and fuel cells. 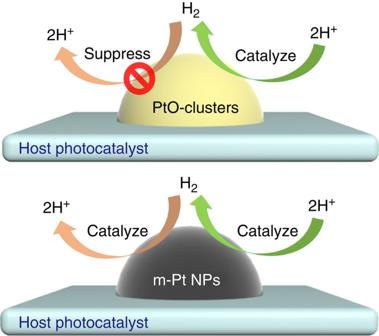Figure 1: Schematic photocatalytic H2evolution and back-reaction processes. Both PtO-clusters and metallic Pt nanoparticles (m-Pt NPs) cocatalysts can act as H2evolution site on host photocatalyst surface, whereas the undesirable H2back-reaction can be suppressed by PtO-clusters cocatalyst but facilitated by m-Pt NPs cocatalyst. Figure 1: Schematic photocatalytic H 2 evolution and back-reaction processes. Both PtO-clusters and metallic Pt nanoparticles (m-Pt NPs) cocatalysts can act as H 2 evolution site on host photocatalyst surface, whereas the undesirable H 2 back-reaction can be suppressed by PtO-clusters cocatalyst but facilitated by m-Pt NPs cocatalyst. Full size image Loading cocatalysts In a typical cocatalyst loading process, the metallic Pt was loaded on anatase TiO 2 {001} nanosheets ( Supplementary Fig. S1 ) through conventional chemical reduction (CCR) method [17] , which used sodium borohydride (NaBH 4 ) as reductant that can readily reduce Pt 4+ precursor into m-Pt NPs (denoted as Pt/TiO 2 ). On the basis of CCR process, poly(methacrylic acid) ligands; (see Supplementary Note 1 for details; Supplementary Figs S2 and S3 ) were involved in ligands-assist chemical reduction (LCR) process, which can controllably load pure PtO-clusters cocatalyst with ultrafine particle size and extraordinary stability on the same TiO 2 {001} nanosheets (denoted as PtO/TiO 2 ; see Methods for detailed experimental method). The Pt loading amount of the as-prepared photocatalysts can be tested to be 1.0 wt% for Pt/TiO 2 and 0.5 wt% for PtO/TiO 2 by inductively coupled plasma (ICP)-atomic emission spectroscopy. Electron microscopy The geometric morphology of the initial PtO/TiO 2 photocatalyst was first examined by high-resolution transmission electron microscopy (TEM). As illustrated in Supplementary Fig. S4 , the photocatalyst has a clean surface and the particle size of the current PtO-clusters (white circles) is extreme small. Interestingly, no apparent diffraction rings of PtO can be observed in selected-area electron diffraction pattern, whereas all diffraction rings can correspond to the host TiO 2 photocatalyst [18] , which may owe to the small size and loading amount of the PtO-clusters cocatalyst. Meanwhile, it can be clearly found that the isolated PtO-clusters (bright spots) are uniformly dispersed on TiO 2 surface, as shown in the scanning TEM image (STEM; Fig. 2a ), and the particle size distribution of the PtO-clusters (inset of Fig. 2a ) reflects that the LCR process can optimize the cocatalyst to be subnanometre-sized cluster, whereas the CCR process demonstrates uncontrollable loading results that show disordered morphology of metallic Pt cocatalyst with a mean particle size around 2 nm ( Supplementary Fig. S5 ). The PtO-clusters are well dispersed over the basal planes and edges of the TiO 2 {001} nanosheets, possibly originating from the strong interactions between the surface functional groups and ligand-assisted Pt ions, and subsequently the formation of oxidized Pt. Specifically, according to the STEM characterization, the PtO-cluster is found to usually contain 6~10 Pt atoms. 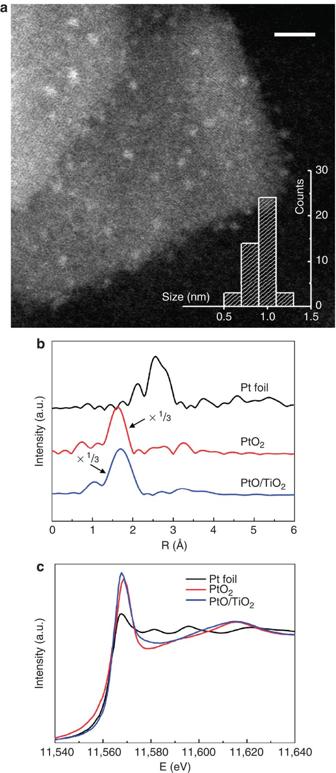Figure 2: Structure analyses of initial PtO/TiO2photocatalytic system. (a) Representative STEM image where isolated three-dimensional PtO-clusters (bright spots) can be observed clearly. The particle size distribution of PtO-clusters cocatalyst is shown in the inset, and the average particle size as estimated from STEM image is 1.0±0.3 nm. Scale bar, 5 nm. (b) The k3-weighted Fourier transform spectra from EXAFS. ×13represents signal magnification. (c) The normalized X-ray absorption near-edge structure spectra at the Pt L3-edge of the Pt foil, PtO2and initial PtO/TiO2photocatalyst. Figure 2: Structure analyses of initial PtO/TiO 2 photocatalytic system. ( a ) Representative STEM image where isolated three-dimensional PtO-clusters (bright spots) can be observed clearly. The particle size distribution of PtO-clusters cocatalyst is shown in the inset, and the average particle size as estimated from STEM image is 1.0±0.3 nm. Scale bar, 5 nm. ( b ) The k 3 -weighted Fourier transform spectra from EXAFS. × 1 3 represents signal magnification. ( c ) The normalized X-ray absorption near-edge structure spectra at the Pt L 3 -edge of the Pt foil, PtO 2 and initial PtO/TiO 2 photocatalyst. Full size image X-ray photoelectron spectroscopy To examine the chemical state and dispersion of Pt species in both cocatalysts, the PtO/TiO 2 and Pt/TiO 2 photocatalysts were then studied by X-ray photoelectron spectroscopy (XPS; Supplementary Fig. S6 ). The main peaks in PtO/TiO 2 photocatalyst centre at 72.4 and 75.8 eV, which can be assigned to Pt 2+ bonded to oxygen [19] . On the other hand, Pt/TiO 2 photocatalyst has two obvious peaks of Pt 4 f 7/2 and 4 f 5/2 at 70.9 and 74.3 eV, respectively, indicating the existence of the metallic Pt. However, the existence of PtO 2 phase can be safely ruled out because the binding energies of Pt 4+ 4 f 7/2 and 4 f 5/2 are 73.8 and 77.1 eV, respectively [20] . Thus, the Pt species in PtO/TiO 2 and Pt/TiO 2 photocatalysts are assigned to PtO and metallic Pt, respectively. Specifically, the dispersion of Pt in both photocatalysts can be evaluated by the relative XPS intensity ratio of Pt atom to Ti atom ( I Pt / I Ti ; Supplementary Table S1 ). On the basis of the initial ICP result discussed above, the high value of I Pt / I Ti in PtO/TiO 2 (0.021) demonstrates the excellent dispersion of PtO-clusters on TiO 2 surface, and the low value of I Pt / I Ti in Pt/TiO 2 (0.014) might be caused by the average particle size of metallic Pt that significantly exceeds the electron escape depth [21] . Moreover, XPS analysis suggests that the O 1 s and Ti 2 p in two photocatalysts are quite similar ( Supplementary Figs S7 and S8 ), indicating that no conspicuous affection occurred on the surface atomic structures of the host TiO 2 during the cocatalyst loading process. Further, according to high-resolution TEM and XPS analysis, no ligands can be detected in the PtO/TiO 2 photocatalyst, indicating that the ligands used in LCR process have been completely removed in washing process through the strong intermolecular force with ethanol. X-ray absorption fine structure studies Fourier-transformed spectrum of the Pt L 3 -edge extended X-ray absorption fine structure (EXAFS) for the PtO/TiO 2 photocatalyst is displayed in Fig. 2b , which shows only one apparent peak at 1.0–2.0 Å. To identify the nature of the backscatterer, EXAFS spectra of Pt and PtO 2 samples were measured as reference. The peak at 1.0–2.0 Å in PtO 2 is because of scattering from the nearest oxygen atoms, whereas the peak at 2.0–3.3 Å in Pt foil is because of scattering from the neighbouring Pt. Thus, the only peak at 1.0–2.0 Å in PtO/TiO 2 is believed to be the contribution from Pt-O binding. Owing to the high disordering in the higher shells, only the main peak in the R ranging from 1.0 to 2.0 Å was considered in the EXAFS curve-fitting (fitting parameters are shown in Supplementary Table S2 ). There is Pt-O contribution at a distance of 2.07 Å for the PtO/TiO 2 photocatalyst, and the coordination number is 4.0, suggesting the Pt species is the PtO phase, which agrees well with the literature data [22] . Figure 2c shows the normalized X-ray absorption near-edge structure spectrum of PtO/TiO 2 photocatalyst, and the reference spectra of Pt foil and PtO 2 . The white-line intensities in the spectra reflect the oxidation state of Pt in different samples. Thus, the white-line intensity of the PtO/TiO 2 , which is close to that of PtO 2 , further suggests that the Pt in the photocatalyst exists as oxidized Pt. Combined with XPS analysis, it can be concluded that the Pt species in the photocatalyst is the PtO phase. HOR suppression ability of the PtO-clusters HOR suppression ability was measured over the as-prepared Pt/TiO 2 and PtO/TiO 2 photocatalysts. In a typical experiment, 50 mg of either photocatalyst was dispersed in 100 ml of deionized water in the reaction vessel. H 2 (2 ml) and O 2 (1 ml) with stoichiometric composition were injected into the closed system before the photocatalytic H 2 evolution test; the gas content was monitored every 15 min via an online gas chromatograph ( Fig. 3a ). Interestingly, a remarkable decrease of both H 2 and O 2 amount was observed on Pt/TiO 2 photocatalyst, which exhibits negligible photocatalytic activity for pure water splitting even after extended periods of light irradiation, mainly because of the rapid undesirable HOR on m-Pt NPs cocatalyst. However, photocatalyst loaded with the PtO-clusters gave stoichiometric H 2 and O 2 evolution from pure water under ultraviolet–visibile light irradiation. Both H 2 and O 2 evolve steadily and stoichiometrically as the reaction proceeds, indicating that the PtO-clusters cocatalyst demonstrates a remarkable HOR suppression capability. It should be noticed that the photogenerated holes may react with TiO 2 and water to form peroxotitanate complexes at the surface and H 2 O 2 in solution [23] . Thus, a photocatalytic test in pure water (100 ml) without adding H 2 and O 2 in the reactor was performed to further confirm the molecular O 2 evolution ( Supplementary Fig. S9 ). The stoichiometric H 2 and O 2 still evolve steadily as the reaction proceeds, indicating that the molecular O 2 (together with H 2 ) can be evolved in the gas phase through pure water splitting in the current PtO/TiO 2 photocatalytic system. Moreover, the HOR suppression ability was also measured in darkness ( Supplementary Fig. S10 ). A similar decrease of both H 2 and O 2 amount was observed on Pt/TiO 2 photocatalyst, whereas the HOR on PtO/TiO 2 was negligible. Thus, it is clear that water formation from H 2 and O 2 on m-Pt NPs is significant during water-splitting reaction. However, in the PtO/TiO 2 photocatalytic system, the suppression of water formation is significant, which is essential to achieve efficient evolution of H 2 and O 2 . 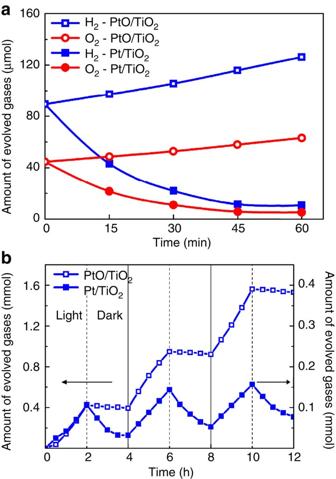Figure 3: HOR suppression in photocatalytic H2evolution test. (a) Reaction time profiles of the HOR with H2and O2on PtO/TiO2and Pt/TiO2photocatalysts under ultraviolet–visible light irradiation (λ>300 nm). In a typical experiment, 2 ml of H2and 1 ml of O2were injected into the evacuated system with the time set as 0. (b) H2evolution and undesirable oxidation in methanol aqueous solution under ultraviolet–visible light irradiation (λ>300 nm, 2 h) and followed dark condition (light off, 2 h) for three times on PtO/TiO2and Pt/TiO2. PtO/TiO2: 219.3 μmol h−1(light),−16.0 μmol h−1(dark); Pt/TiO2: 53.8 μmol h−1(light),−41.0 μmol h−1(dark). Figure 3: HOR suppression in photocatalytic H 2 evolution test. ( a ) Reaction time profiles of the HOR with H 2 and O 2 on PtO/TiO 2 and Pt/TiO 2 photocatalysts under ultraviolet–visible light irradiation ( λ >300 nm). In a typical experiment, 2 ml of H 2 and 1 ml of O 2 were injected into the evacuated system with the time set as 0. ( b ) H 2 evolution and undesirable oxidation in methanol aqueous solution under ultraviolet–visible light irradiation ( λ >300 nm, 2 h) and followed dark condition (light off, 2 h) for three times on PtO/TiO 2 and Pt/TiO 2 . PtO/TiO 2 : 219.3 μmol h −1 (light), − 16.0 μmol h −1 (dark); Pt/TiO 2 : 53.8 μmol h −1 (light), − 41.0 μmol h −1 (dark). Full size image In addition, the HOR suppression abilities of both photocatalysts were also studied in methanol aqueous solution (100 ml, 30 v/v %). The reaction vessel was initially irradiated for 2 h (light reaction), and then kept in darkness for another 2 h (dark reaction) to observe the H 2 back-reaction. The amounts of H 2 are illustrated in Fig. 3b . In the light reaction, the photocatalytic H 2 evolution activity of PtO/TiO 2 is nearly four times higher than that of Pt/TiO 2 , which may be attributed to the ultrafine particle size and high dispersion of PtO-clusters compared with that of m-Pt NPs loaded on TiO 2 . Interestingly, in the dark reaction, the pressures of H 2 on the Pt/TiO 2 photocatalyst decreased very quickly, whereas those on PtO/TiO 2 decreased negligibly, which show the same tendencies with respect to the results in pure water system. The inactivity of the PtO-clusters cocatalyst for the undesirable H 2 back-reaction can be a positive characteristic for photocatalytic H 2 generation. The reaction rate ratio of H 2 decrease (dark reaction) to H 2 evolution (light reaction) on PtO/TiO 2 photocatalyst is merely 10 %, whereas that on Pt/TiO 2 drastically climbs to 80 %. Accordingly, in the current PtO/TiO 2 photocatalytic system, the PtO-clusters cocatalyst does govern the favourite direction of H 2 reactions, and can be considered to have two roles: (i) acting as efficient H 2 evolution sites on host photocatalyst surface and (ii) suppressing the undesirable H 2 back-reaction. Photochemical stability as well as photocatalytic activity is crucial factor for a practical photocatalyst. The conventional oxidized Pt species can be reduced to metallic Pt by the photoexcited electrons during photocatalytic tests, especially in methanol aqueous solution [24] , [25] . Therefore, the structure of PtO/TiO 2 photocatalyst was again studied by STEM, XPS and EXAFS analyses after photocatalytic test in methanol aqueous solution. The geometric morphology of PtO/TiO 2 photocatalyst ( Supplementary Fig. S11 ) still exhibits subnanometre PtO-clusters attached on the host photocatalyst surface, suggesting that the isolated PtO-cluster retains excellent structure stability. Moreover, the Pt 4 f XPS spectra and the I Pt / I Ti were detected with negligible difference between the initial and used PtO/TiO 2 photocatalyst ( Supplementary Fig. S12 and Supplementary Table S1 ), and the EXAFS spectra show that the used photocatalyst still has only one apparent peak at 1.0–2.0 Å, suggesting that the Pt species in the used photocatalyst remains as the PtO phase ( Supplementary Fig. S13 ). In addition, the life cycle measurement in methanol aqueous solution was carried out to confirm the photocatalytic stability of the PtO/TiO 2 photocatalyst ( Supplementary Fig. S14 ). The PtO/TiO 2 showed good durability for 6 days of operation under ultraviolet–visible light irradiation. Further, the stability of the PtO/TiO 2 photocatalyst was also explored by virtue of density functional theory (DFT) calculations ( Supplementary Figs S15 and S16 , Supplementary Table S3 ). All results strongly suggest that PtO-clusters cocatalyst we prepared has an excellent stability. DFT studies To demonstrate the relative activity of the oxidized PtO species and metallic Pt cocatalyst in affecting HOR, we investigated the detailed pathways of H 2 reacting with O 2 (H 2 +1/2O 2 →H 2 O) occurring on these two kinds of catalysts by virtue of DFT calculations (see calculation details in Methods). To simulate the oxidized PtO-clusters cocatalyst, Pt 8 O 8 -cluster supported by TiO 2 (001) surface (Pt 8 O 8 /TiO 2 ) was selected on the account of the experimental STEM characterization ( Fig. 2a ), which indicates the PtO cluster usually containing 6~10 Pt atoms, whereas for the metallic Pt cluster on TiO 2 (001) surface, Pt 12 cluster (Pt 12 /TiO 2 ) was tested and selected (see details in Supplementary Table S4 ), in which the molecular dynamics simulation was applied to screen the optimal structure ( Fig. 4a–c ). The common elementary reaction steps involved in HOR on metal Pt surfaces contain (i) adsorption and dissociation of H 2 and O 2 molecule and (ii) the surface O* reacting with H* into OH*, and further to H 2 O. Alternatively, the formation of surface OH* could be accomplished through surface O* reacting with one H 2 O molecule, instead of the direct coupling of surface H* and O* atoms [26] , [27] . As shown in Table 1 , reaction barriers and Gibbs free energy changes of these elementary steps on both Pt 12 /TiO 2 and Pt 8 O 8 /TiO 2 were calculated (see structures in Supplementary Figs S17–S20 and adsorption energies in Supplementary Table S4 ). On Pt 12 /TiO 2 , it is found that O 2 molecule has a large adsorption energy of −1.67 eV (with the gas-phase entropy of O 2 at 298 K included), and the adsorbed O 2 * can easily dissociate into two atomic O* with a large energy gain of 1.51 eV and a barrier as low as 0.49 eV. Meanwhile, H 2 molecule can even directly dissociate into atomic H* on adsorption at Pt 12 /TiO 2 with a large Gibbs free energy gain of 1.06 eV. Therefore, it can be concluded that H 2 and O 2 can be easily activated in the presence of metallic Pt cocatalyst. By contrast, molecular adsorption and activation of O 2 and H 2 on Pt 8 O 8 /TiO 2 become relatively difficult to occur. First, the adsorption of H 2 and O 2 on Pt 8 O 8 /TiO 2 is found to be much weaker, giving a value of 0.14 and 0.34 eV in terms of Gibbs free energy change, respectively. Second, their corresponding dissociations become difficult, being exothermic by only −0.13 eV (O 2 +2*→2O*) and even endothermic by 0.02 eV (H 2 +2*→2 H*). More importantly, the dissociation barriers of O 2 * and H 2 * on Pt 8 O 8 /TiO 2 are also evidently increased to 0.62 eV and 0.17 eV, respectively, indicating that activation of O 2 /H 2 to generate surface H* and O* should be much more difficult on the Pt-oxide compared with metallic Pt cluster on TiO 2 (001) surface. Thus, PtO-clusters cocatalyst presents a higher suppression ability relative to Pt-clusters in decomposing the evolved H 2 into H + and e − reversely or activating the O 2 molecule, which is consistent with the experimental observation shown in Fig. 3 . 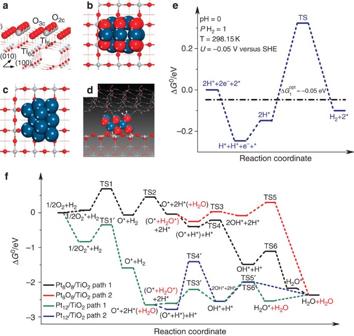Figure 4: Optimized structures and Gibbs free energy profiles. (a) Structure of anatase TiO2(001) surface. (b) Optimized Pt8O8-cluster adsorbed on TiO2(001) surface and (c) optimized Pt12/TiO2. (d) Transition state structure of H*–H* coupling on Pt8O8/TiO2in liquid phase, which contains two layers of water molecules above the Pt8O8-cluster. (e) Standard Gibbs free energy profile of HER in aqueous solution on Pt8O8/TiO2. (f) Standard Gibbs free energy profile of H2reacting with O2on Pt8O8/TiO2and Pt12/TiO2surfaces in gas phase. Dark blue balls represent Pt atoms, grey for Ti, white for H and red for O. Figure 4: Optimized structures and Gibbs free energy profiles. ( a ) Structure of anatase TiO 2 (001) surface. ( b ) Optimized Pt 8 O 8 -cluster adsorbed on TiO 2 (001) surface and ( c ) optimized Pt 12 /TiO 2 . ( d ) Transition state structure of H*–H* coupling on Pt 8 O 8 /TiO 2 in liquid phase, which contains two layers of water molecules above the Pt 8 O 8 -cluster. ( e ) Standard Gibbs free energy profile of HER in aqueous solution on Pt 8 O 8 /TiO 2 . ( f ) Standard Gibbs free energy profile of H 2 reacting with O 2 on Pt 8 O 8 /TiO 2 and Pt 12 /TiO 2 surfaces in gas phase. Dark blue balls represent Pt atoms, grey for Ti, white for H and red for O. Full size image Table 1 Reaction barriers and free energies*. Full size table To be systematic, the full reaction pathways of H 2 O formation from the surface H* and O* catalysed by Pt 12 − and Pt 8 O 8 /TiO 2 were further investigated and compared. With respect to the formation of OH*, it is noteworthy that direct coupling of surface O* and H* to form OH* on Pt 12 /TiO 2 needs to overcome a high barrier of 1.38 eV. Instead, OH* could be generated alternatively through O* reacting with an adsorbed H 2 O* molecule (H 2 O*+O*→2OH*), which has a much lower barrier (0.40 eV), whereas for OH formation on Pt 8 O 8 , this alternative pathway does not give evident facilitation because of an increased barrier of 0.28 eV relative to that (0.19 eV) in the direct O*–H* coupling. In other words, the OH* formation at Pt 8 O 8 /TiO 2 and Pt 12 /TiO 2 could be achieved through different pathways, with the former being easier to occur (0.19 versus 0.40 eV; Fig. 4f ). Further, the corresponding reaction barrier of OH* reacting with H* to form H 2 O on Pt 8 O 8 /TiO 2 is calculated to be 0.38 eV, being a little smaller than that (0.56 eV) on Pt 12 /TiO 2 . Overall, the step of surface intermediates H* and O* transforming into H 2 O is easier to occur on Pt 8 O 8 /TiO 2 surface, in principle rationalized by the weak binding of H* and O* with the oxidized Pt. Nevertheless, from the Gibbs free energy profile of H 2 oxidation by O 2 on Pt 8 O 8 /TiO 2 and Pt 12 /TiO 2 ( Fig. 4f ), one can see that the whole profile on Pt 12 /TiO 2 is entirely below the initial state of the reactants, and also the profile on Pt 8 O 8 /TiO 2 . Specifically, one can see that the rate-determining step in the whole process of both catalysts appears in the dissociation of O 2 based on the kinetic estimation, and the highest point (at the transition state of O 2 dissociation) in the favoured pathway on Pt 8 O 8 (black line) is evidently higher than that of Pt 12 (olive line) with a difference of ~1 eV. Therefore, it can be understood that the reverse formation of H 2 O through H 2 reacting with O 2 is favoured on metallic Pt-clusters; by contrast, H 2 oxidation can be efficiently suppressed on the oxidized PtO-clusters in the dark reaction because of the weak adsorption and dissociation ability of PtO-cluster towards O 2 and H 2 in principle. Further, to confirm the reactivity of the H 2 back-reaction in methanol aqueous solution, DFT calculation was also carried out to demonstrate the relative suppressing ability of the oxidized Pt cluster and metallic Pt NPs (see details in Supplementary Fig. S21 ). Together with the ‘H 2 +1/2O 2 →H 2 O’ reaction addressed above, it can be concluded that no matter which form of possible back reactions, that is, ‘1/2 H 2 →H + +e − ’, ‘H 2 +1/2O 2 →H 2 O’ or ‘H 2 +HCHO→CH 3 OH’, the oxidized Pt 8 O 8 cocatalyst exhibits a remarkable suppressing ability owing to the relatively difficult activation and dissociation of H 2 molecule. In addition to the suppressing ability towards reverse reaction, the catalytic activity of the oxidized Pt species in catalysing HER (H + (aq) +e − +*→1/2 H 2 ) was also approximately estimated within the thermodynamics framework. By performing DFT calculation, thermodynamics of each elementary step of HER occurring on Pt 8 O 8 /TiO 2 in the water environment was calculated, in which the standard hydrogen electrode (SHE) was used as the reference to calculate the Gibbs free energy change (Δ G ) of HER (see details in Methods). It indicated that there exists a volcano-shaped relation between the catalytic activity of HER and the Gibbs free energy change (Δ G 1 ) of the proton adsorption step (H + (aq) +e − +*→H*) by applying the basic thermodynamic model [28] , and our recent work showed that the maximum reaction rate of HER occurring on Pt(O)/TiO 2 catalysts could be arrived at the point of Δ G 1 opt =−0.05 eV (unpublished results), which means Δ G 1 can be utilized as a measurement. On Pt 8 O 8 /TiO 2 , Δ G 1 for the proton adsorption process were calculated to be −0.25 and 0.10 eV for the first and the second proton adsorption, respectively (see details in Supplementary Fig. S22 and Supplementary Table S5 ), both of which are close to the optimal adsorption strength (Δ G 1 opt =−0.05 eV). Interestingly, Δ G 2 (2 H*→H 2 +2*) was only 0.05 eV, showing the thermodynamic easiness of H* coupling into H 2 . Further, we tried to locate the transition state for H*–H* coupling reaction ( Fig. 4d ), giving a reaction barrier as low as 0.47 eV. The standard Gibbs free energy profile of HER on Pt 8 O 8 /TiO 2 in the aqueous solution is illustrated in Fig. 4e , from which one can see that there is no evidently high point in the whole profile, suggesting the excellent performance of the oxidized Pt species (Pt 8 O 8 ) in catalysing HER. In summary, PtO-clusters were found to have a pivotal role in unidirectional suppression of undesirable H 2 oxidation in photocatalytic water cleavage process. More importantly, these PtO-clusters can also demonstrate excellent efficiency in hydrogen evolution rate. Quantum chemical calculations have been applied to rationalize these experimentally observed structure–performance relations, and the origin of the promising performance of the oxidized Pt species in catalysing HER as well as suppressing unfavourable H 2 oxidation was also revealed. On the basis of experimental findings and theoretical models in this work, other high-efficient heterogeneous catalysts or catalytic systems might be developed for clean energy and environment applications. Fabrication of photocatalysts The TiO 2 {001} nanosheets and poly(methacrylic acid) polymer ligands were synthesized according to the literatures [29] , [30] . For PtO/TiO 2 photocatalyst, 50 mg of TiO 2 and 24.6 mg of polymer ligands were added into a screw-neck glass bottle (10 ml) containing chloroplatinic acid solution (5 ml, 0.2 mg ml −1 ). After the solution becoming uniform by sonication, 0.5 ml of freshly prepared NaBH 4 aqueous solution (2 mg ml −1 ) was rapidly injected into the solution under vigorous stirring (2,000 r.p.m.). After 2~3 h, another 0.5 ml of freshly prepared NaBH 4 solution was injected into the solution again. The stirring speed of the solution was kept at the same 2,000 r.p.m. for >10 h. In the washing process, the precipitate was sonicated for >2 min every time to ensure all photocatalyst dispersing uniformly in cleaning solution, and then separated by centrifuge. The precipitate was washed by deionized water for three times and ethanol for five times. After dried at room temperature, PtO/TiO 2 photocatalyst with clean surface was collected. The Pt/TiO 2 photocatalyst was synthesized using the similar process without adding the polymer ligands. Photocatalysts characterization The crystal structure was determined using X-ray diffraction (Bruker D8 Advanced Diffractometer with Cu K α radiation). The molecular weight distribution of polymer ligands was measured by gel permeation chromatography (Waters). The detailed structural information of polymer ligands were analysed by Fourier transform infrared spectroscopy (Nicolet 5700) and NMR (Avance, 400 MHz) measurements. The loading amount of the cocatalysts was tested by ICP-atomic emission spectroscopy (Varian 710 ES). Further, the structure of the photocatalysts was examined by TEM (Tecnai 30, 300 kV). The chemical states of the elements in two photocatalytic systems were studied by XPS (Kratos Axis Ultra DLD), and the binding energy of the C 1 s peak at 284.8 eV was taken as an internal reference. Pt L 3 -edge absorption spectra (EXAFS) were performed on the 1W2B beamline of the Beijing Synchrotron Radiation Facility, China, operated at ~200 mA and ~2.5 GeV. Pt foil and PtO 2 were used as reference samples and measured in the transmission mode, and the initial and used PtO/TiO 2 photocatalysts were measured in fluorescence mode. We used IFEFFIT software to calibrate the energy scale, to correct the background signal and to normalize the intensity. Photocatalytic H 2 evolution test The photocatalytic H 2 evolution test was carried out in a glass gas-closed-circulation system with a top irradiation-type reaction vessel (LabSolar H 2 ) and a 300-W xenon lamp (CEL-HXBF300). The temperature of reactant solution was maintained at 20 o C by a flow of cooling water during the test. Fifty milligrams of photocatalyst dispersed in solvent were added into the reaction vessel for photocatalytic H 2 evolution test. The amounts of evolved H 2 and O 2 were monitored by an online gas chromatograph (GC7890T). No air should be present in the system after evacuation by vacuum pump. Theoretical calculation All the spin-polarized calculations were performed with Perdew–Burke–Ernzerhof functional [31] within the generalized gradient approximation, in which the VASP package was used [32] , [33] . The project-augmented wave method was used to represent the core-valence electron interaction [34] , [35] . To model the anatase TiO 2 (001) surface, a three-layer p (2 × 2) slab (10.772 × 10.772 Å 2 ) corresponding to 48 TiO 2 units cell (144 atoms) was used, in which a vacuum layer of 15 Å was applied and the top layer of TiO 2 was allowed to relax. Because of the large size of the supercell, Monkhorst Pack mesh with Γ point k -point sampling in the surface Brillouin zone was used. For total energy calculations, the valence electronic states were expanded in plane wave basis sets with a cutoff energy of 450 eV. Atomic positions were relaxed until the absolute forces of each atom were <0.05 eV/Å. Free energy calculation method In the reaction of proton adsorbing and receiving excited electron, the proton–electron pair is always involved simultaneously in photocatalytic process. To obtain the free energy of the each elementary step, when involving H + +e – , the SHE was used as the reference in standard Gibbs free energy calculation of HER [28] . Gibbs free energy changes of step (i) H + (aq) +e – +*→H* and (ii) 2 H*→H 2 +2* (corresponding to Δ G 1 and Δ G 2 , respectively) can be calculated as follows: in which U is the electronic voltage of an excited electron versus SHE (here it is at the conduction band bottom of anatase TiO 2 ), and therefore e U equals to −0.05 eV, whereas P H 2 and C H + are the relative partial pressure of H 2 in gas phase and the relative concentration of H + in the aqueous solution, respectively (see more details in Supplementary Note 3 ). The adsorption energy ( E ad H ) for H 2 was obtained from the DFT calculation at 0 K relative to the gas-phase H 2 molecule, which is defined as where E H/sur , E sur and E H 2 are the total energy of the adsorption system, the clean surface and the H 2 molecule, respectively. How to cite this article: Li, Y. H. et al . Unidirectional suppression of hydrogen oxidation on oxidized platinum cluster. Nat. Commun. 4:2500 doi: 10.1038/ncomms3500 (2013).